Caste-specific RNA editomes in the leaf-cutting antAcromyrmex echinatior Eusocial insects have evolved the capacity to generate adults with distinct morphological, reproductive and behavioural phenotypes from the same genome. Recent studies suggest that RNA editing might enhance the diversity of gene products at the post-transcriptional level, particularly to induce functional changes in the nervous system. Using head samples from the leaf-cutting ant Acromyrmex echinatior , we compare RNA editomes across eusocial castes, identifying ca . 11,000 RNA editing sites in gynes, large workers and small workers. Those editing sites map to 800 genes functionally enriched for neurotransmission, circadian rhythm, temperature response, RNA splicing and carboxylic acid biosynthesis. Most A. echinatior editing sites are species specific, but 8–23% are conserved across ant subfamilies and likely to have been important for the evolution of eusociality in ants. The level of editing varies for the same site between castes, suggesting that RNA editing might be a general mechanism that shapes caste behaviour in ants. Ants have highly organized eusocial colonies consisting of morphologically differentiated castes that specialize in egg-laying (queens) or non-reproductive functions such as nursing, nest-building, foraging and defense (workers and occasionally soldiers) [1] . Caste phenotypes represent distinct developmental pathways that are plastic during early larval development and produce adults that vary in size, physiology, life span and behaviour [1] , [2] , [3] . Previous studies have suggested that epigenetic factors may be more important for caste differentiation than originally appreciated [4] , [5] . Recent studies in honeybees and ants have also uncovered details of differential gene expression, DNA methylation and histone modification associated with profound behavioural differences between eusocial castes [6] , [7] , [8] , [9] . However, post-transcriptional gene regulation via RNA editing has remained unexplored in social insects, in spite of its known importance for nervous system functions [10] , [11] that have been documented in model species such as nematodes [12] , [13] , fruit flies [14] , [15] , mice [16] and humans [17] , [18] , [19] , [20] . RNA editing alters RNA sequences through individual base substitutions, insertions or deletions, and thus enhances gene product diversity [21] , [22] . The most prevalent type of RNA editing in the animal kingdom is A-to-I editing, where adenosine (A) residues are converted to inosine (I) catalysed by adenosine deaminase (ADAR) enzymes that use double-stranded RNAs (dsRNAs) as substrate [22] . As inosine is recognized as guanosine by the ribosome during translation, A-to-I editing in protein-coding sequences may result in amino acid changes that alter the functional properties of proteins [22] . A-to-I editing can also play an important role in regulating gene expression by affecting alternative splicing [23] , editing microRNA (miRNA) sequences [24] or changing miRNA target sites in messenger RNA [25] . Drosophila with an ADAR -null mutation preventing A-to-I editing exhibit severe behavioural and locomotory abnormalities [11] , while Caenorhabditis elegans with homozygous deletions of both adr-1 and adr-2 show chemosensory defects [12] . The effects of preventing RNA editing in mammals are even more striking. Adar1 −/− mice die in the embryonic stage [26] and Adar2 −/− mice suffer profound epileptic seizures and die shortly after birth [27] . The recent application of next-generation sequencing technology has greatly facilitated the genome-wide detection of RNA editing events and demonstrated that RNA editing of genomic information is pervasive [13] , [14] , [15] , [16] , [17] , [18] , [19] , [20] . RNA editing appears to frequently target transcripts that encode proteins involved in the propagation of fast electrical and chemical signals in animal nervous systems, such as voltage-gated ion channels, ligand-gated receptors and key components of the pre-synaptic release machinery [10] . This was recently confirmed by a study in octopuses, which showed that levels of RNA editing were associated with the function of K + channels mediating adaptation to temperature change [28] . As the nervous systems coordinate animal behaviours in response to both internal and external stimuli [29] , there are multiple reasons to expect that RNA editing of genes expressed in the nervous systems of eusocial insects might provide an important regulatory mechanism for behavioural differences among eusocial castes. We used the leaf-cutting ant Acromyrmex echinatior to investigate the characteristics and putative roles of RNA editing in eusocial insects. This ant species has three female castes: small workers, large workers and queens (referred to as gynes when still winged and unmated). A. echinatior belongs to the crown group of the attine fungus-growing ants [30] and has the peculiar characteristics associated with this group, such as a diet almost exclusively derived from a specialized fungus-garden symbiont, foraging on fresh leaves that are processed in a conveyor-belt manner and additional symbioses with antibiotic-producing bacteria [31] . We recently sequenced the genome of A. echinatior and produced a high-quality assembled and annotated draft genome [32] , which provided us with the opportunity to further investigate possible genome-wide mechanisms of caste differentiation. Here we use strand-specific RNA-Seq on head tissue samples of the female castes of A. echinatior and data from other genome-sequenced ants to evaluate the possible role of RNA editing in modulating functional gene differentiation among castes, and show that RNA editing may be an important but underappreciated mechanism that shapes caste behaviour in ants. Enzymes responsible for RNA editing Vertebrate genomes are known to contain at least three ADAR genes ( ADAR1 , ADAR2 and ADAR3 ) and two of these ( ADAR1 and ADAR2 ) have been confirmed to be also present in invertebrate genomes, including a sea anemone ( Nematostella vectensis ), an oyster ( Crassostrea gigas ), a sea urchin ( Strongylocentrotus purpuratus ) and a tunicate ( Ciona intestinalis ) [33] . However, the genome of A. echinatior encodes only a single ADAR gene, but with two dsRNA-binding domains and one deaminase domain it appears more similar to ADAR2 than ADAR1 in other animals ( Fig. 1a and Supplementary Fig. 1a ). This finding is consistent with previous observations in other insects [33] and supports the view that the common ancestor of the insects lost ADAR1 . Gene structures and protein sequences of ADAR genes were highly conserved among 11 different ant species for which sequenced genomes were available, indicating that selection on this gene has been severely constrained ( Fig. 1b and Supplementary Fig. 1b ). We found that ADAR was widely expressed across the different castes of A. echinatior and two other ants ( Camponotus floridanus and Harpegnathos saltator ), and across different developmental stages of C. floridanus and H. saltator ( Fig. 1c and Supplementary Fig. 2a,b ), indicating that A-to-I RNA editing is likely to be operational throughout the life cycles of ants. We further observed that the expression levels of ADAR in small A. echinatior workers were higher than in gynes and large workers ( Fig. 1c and Supplementary Fig. 2c,d ). 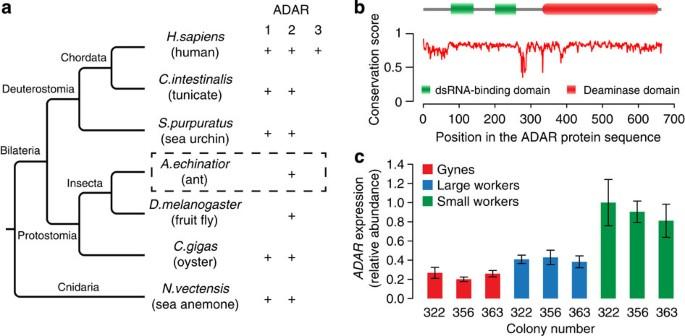Figure 1:ADARin the leaf-cutting antA. echinatiorand other sequenced genomes. (a) Variation in the number ofADARgenes across animals, showing that the insect lineage, includingA. echinatior, has lostADAR1but preservedADAR2. (b) Domain organization and conservation scores of the ADAR protein sequences in ants, showing thatADAR2is highly conserved during ant evolution. Conservation scores were calculated from the multiple sequence alignments of the ADAR protein sequences across 11 ant species with sequenced genomes using the Jensen–Shannon divergence method65:A. echinatior,Atta cephalotes,C. floridanus,Pogonomyrmex barbatus,Linepithema humile,H. saltator(http://hymenopteragenome.org/ant_genomes/) and five other attine species (Atta colombica,Trachymyrmex septentrionalis,Trachymyrmex cornetzi,Trachymyrmex zetekiandCyphomyrmex costatus), whose genome sequences were available but not yet published (Nygaardet al, in preparation). (c) Expression levels ofADARdenoted by real-time qPCR in the three female castes ofA. echinatior. The housekeeping geneEf1-betawas chosen as internal reference gene. Error bars are s.d. across the three replicates. Figure 1: ADAR in the leaf-cutting ant A. echinatior and other sequenced genomes. ( a ) Variation in the number of ADAR genes across animals, showing that the insect lineage, including A. echinatior , has lost ADAR1 but preserved ADAR2 . ( b ) Domain organization and conservation scores of the ADAR protein sequences in ants, showing that ADAR2 is highly conserved during ant evolution. Conservation scores were calculated from the multiple sequence alignments of the ADAR protein sequences across 11 ant species with sequenced genomes using the Jensen–Shannon divergence method [65] : A. echinatior , Atta cephalotes , C. floridanus , Pogonomyrmex barbatus , Linepithema humile , H. saltator ( http://hymenopteragenome.org/ant_genomes/ ) and five other attine species ( Atta colombica , Trachymyrmex septentrionalis , Trachymyrmex cornetzi , Trachymyrmex zeteki and Cyphomyrmex costatus ), whose genome sequences were available but not yet published (Nygaard et al , in preparation). ( c ) Expression levels of ADAR denoted by real-time qPCR in the three female castes of A. echinatior . The housekeeping gene Ef1-beta was chosen as internal reference gene. Error bars are s.d. across the three replicates. Full size image In addition to A-to-I editing, a much rarer type of cytosine-to-uracil (C-to-U) RNA editing has also been documented in mammals [34] and fruit flies [35] , and our data also imply the existence of a small number of C-to-U editing sites in A. echinatior (see below). C-to-U RNA editing results from cytosine deamination catalysed by APOBECs (an apolipoprotein B mRNA-editing enzyme with polypeptide-like catalytic function) in mammals [34] , but we have not been able to identify orthologues of these genes in ants or other insects, suggesting that insects use other enzymes with cytidine deaminase activity to perform C-to-U RNA editing. Caste-specific RNA editomes To assess the RNA-editing patterns across different castes, we carried out strand-specific RNA-Seq [36] on polyA+ RNA isolated from adult head tissues of the three female castes of A. echinatior : gynes, large workers and small workers. We sampled three sympatric colonies and sequenced them separately ( Supplementary Table 1 ). To help filtering out possible DNA–RNA differences caused by heterozygous single-nucleotide polymorphisms (SNPs), we also resequenced the DNA isolated from the remaining tissues of exactly the same individuals as used for RNA-Seq (see Methods). On average, we obtained ca . 11 Gb RNA-Seq and ca . 12 Gb DNA-Seq data for each of the nine samples, representing a genome-wide coverage depth of ca . 37 × and 39 × , respectively. After mapping and rigorous filtering (see Methods), we obtained an average usable depth of ca . 11 × for RNA samples and ca . 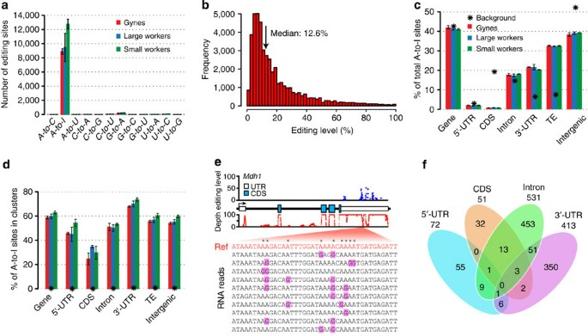Figure 2: RNA-editing sites identified in samples of gynes, large workers and small workers ofA. echinatior. (a) Distribution of the mean number of editing sites across the 12 possible types of RNA editing in each caste-specific sample. (b) Frequency distribution of editing levels for all editing sites with RNA coverage ≥20 × after pooling the editing sites from all nine samples (gynes, large workers and small workers from three colonies; arrow is the median editing level of 12.6%). (c) Percentages of A-to-I editing sites across different genomic elements. Black asterisks indicate the background expectations, which were calculated as the number of transcribed ‘A’s (that is, ‘A’s with RNA-Seq read coverage ≥1 × ) in each genomic element divided by the total number of transcribed ‘A’s in the genome. The ‘Gene’ category is the sum of untranslated regions (5′-UTR and 3′-UTR), CDSs and introns, while the ‘Intergenic’ category represents all genomic regions that are neither genes nor TEs. (d) Percentages of A-to-I editing sites occurring in clusters (≥3 sites within a 50-bp window) across different genomic elements. The same number of transcribed ‘A’s as the identified A-to-I editing sites in each genomic element was randomly selected and used for calculating background expectations (indicated by black asterisks representing values close to zero). (e) RNA editing of the geneMdh1in large workers from colony 322, involving 84 A-to-I editing sites (blue points) in the 3′-UTR of this gene where the editing sites always occur in clusters. (f) Venn diagram of edited genes showing the genic positions of their editing sites. The numbers presented were counted in large workers from colony 322, but the other samples showed similar patterns. Error bars ina,canddare s.d. across the three colonies. 24 × for DNA samples for further analysis ( Supplementary Table 2 ). To identify candidate RNA-editing sites, we designed a statistical framework to detect sites that were homozygous for genomic DNA (gDNA), but heterozygous for transcripts (see Methods). The orientation information provided by strand-specific RNA-Seq then allowed us to determine the RNA–DNA base differences independent of existing genomic annotations. 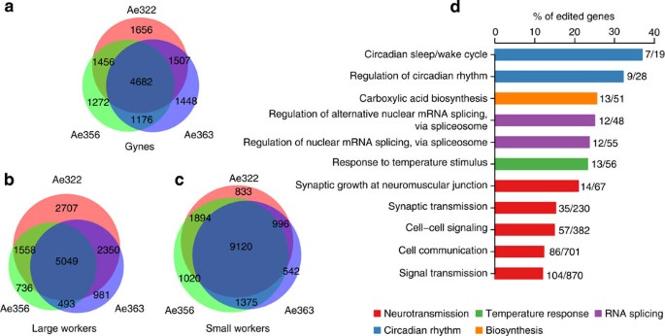Figure 3: Functional editing sites in the leaf-cutting antA. echinatior. (a–c) Venn diagrams of A-to-I editing sites across the three different colonies Ae322, Ae356 and Ae363. (d) Over-represented Gene Ontology (GO) terms for the 835 genes that were consistently edited in at least one caste, showing the percentages of edited genes relative to all transcribed genes annotated to corresponding GO terms. The first number after each bar indicates the number of edited genes annotated to this GO term, and the second number indicates the number of all transcribed genes (RPKM >1 in at least one of the nine sequenced samples) annotated to this GO term. 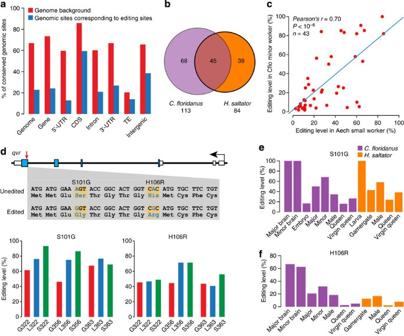Figure 4: Conservation of RNA editing among ant species. (a) Percentage of conserved genomic sites that display the same DNA bases among seven attine ant species. The ‘Gene’ category is the sum of 5′-UTRs, 3′-UTRs, CDSs and introns, and the ‘Intergenic’ category represents all genomic regions that are neither genes nor TEs. The red bars (genome background) were calculated from all transcribed ‘A’s (that is, ‘A’s covered by ≥1 RNA reads) in each category, and the blue bars from genomic sites corresponding to A-to-I RNA editing sites in each category. (b) The number of conserved editing events (sites displaying the same RNA base substitutions among species) betweenA. echinatiorandC. floridanusand betweenA. echinatiorandH. saltator. (c) Correlation of RNA-editing levels for the conserved editing events between heads of small workers ofA. echinatiorand brains of minor workers ofC. floridanus. Only sites with RNA read coverage ≥10 × in both samples were used. Editing levels ofA. echinatiorsmall workers were calculated from the combined data of the three small worker samples. The blue line is a linear regression that is virtually identical to the diagonal. (d) Editing of theqvrgene inA. echinatior. The upper part shows theqvrgene model and the two editing sites, as well as their protein recoding potential. The red arrow in the sixth exon indicates the positions of the two neighbouring editing sites. The lower part shows the editing levels of the two sites in the nine head samples (G, L, S stand for gynes, large workers and small workers, respectively, and are followed by colony number). (e,f) Editing levels of the corresponding sites ofqvrinC. floridanusandH. saltator. We identified an average of 10,715 editing sites (range 8,146–13,823) per sample ( Supplementary Table 3 ), with an average of 969 genes (range 812–1,125) being edited in one or more sites ( Supplementary Table 4 ). As observed in humans [17] , [18] , [19] , [20] , mice [16] and fruit flies [14] , [15] , most (up to 97%) of the editing sites represented A-to-I editing ( Fig. 2a and Supplementary Table 3 ), indicating that non-A-to-I RNA editing is rare in A. echinatior . Figure 2: RNA-editing sites identified in samples of gynes, large workers and small workers of A. echinatior . ( a ) Distribution of the mean number of editing sites across the 12 possible types of RNA editing in each caste-specific sample. ( b ) Frequency distribution of editing levels for all editing sites with RNA coverage ≥20 × after pooling the editing sites from all nine samples (gynes, large workers and small workers from three colonies; arrow is the median editing level of 12.6%). ( c ) Percentages of A-to-I editing sites across different genomic elements. Black asterisks indicate the background expectations, which were calculated as the number of transcribed ‘A’s (that is, ‘A’s with RNA-Seq read coverage ≥1 × ) in each genomic element divided by the total number of transcribed ‘A’s in the genome. The ‘Gene’ category is the sum of untranslated regions (5′-UTR and 3′-UTR), CDSs and introns, while the ‘Intergenic’ category represents all genomic regions that are neither genes nor TEs. ( d ) Percentages of A-to-I editing sites occurring in clusters (≥3 sites within a 50-bp window) across different genomic elements. The same number of transcribed ‘A’s as the identified A-to-I editing sites in each genomic element was randomly selected and used for calculating background expectations (indicated by black asterisks representing values close to zero). ( e ) RNA editing of the gene Mdh1 in large workers from colony 322, involving 84 A-to-I editing sites (blue points) in the 3′-UTR of this gene where the editing sites always occur in clusters. ( f ) Venn diagram of edited genes showing the genic positions of their editing sites. The numbers presented were counted in large workers from colony 322, but the other samples showed similar patterns. Error bars in a , c and d are s.d. across the three colonies. Full size image The median editing level was rather low (12.6%) and only ca . 8% of the editing sites had editing levels (the ratio of RNA-Seq reads with editing versus total RNA reads) over 50% ( Fig. 2b , also see Supplementary Fig. 3 for separating A-to-I and non-A-to-I editing sites). Consistent with the known properties of ADAR enzymes [22] , A-to-I editing sites were concentrated in potentially dsRNA regions, relative to random controls in A. echinatior ( Supplementary Fig. 3c and Supplementary Methods ). Similar to observations in humans [18] , [19] and fruit flies [15] , the A. echinatior bases in upstream and downstream positions adjacent to A-to-I editing sites (−1 and +1 positions) had a deficiency and excess of guanines, respectively ( Supplementary Fig. 3e and Supplementary Methods ). In addition, A-to-I editing sites clearly occurred in clusters ( Fig. 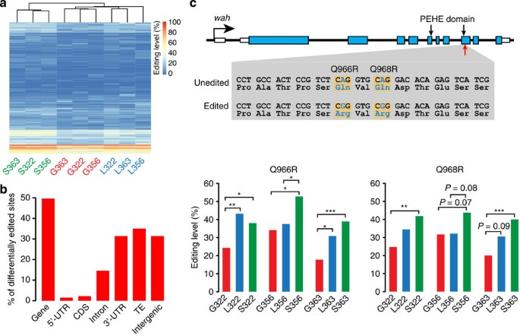Figure 5: Caste-specific RNA editing inA. echinatior. (a) Heatmap and hierarchical clustering based on editing levels of all the editing sites identified in the nine samples (G, L, S stand for gynes, large workers and small workers, respectively, and are followed by colony number). Sites for which editing was confirmed in at least one of the nine samples and that had RNA read depth ≥20 × in all the nine samples were used (n=2,944). (b) Percentages of the 137 consistently differentially edited sites across different genomic elements. The ‘Gene’ category is the sum of 5′-UTRs, 3′-UTRs, CDSs and introns, and the ‘Intergenic’ category represents all genomic regions that are neither genes nor TEs. (c) RNA editing ofwah(Aech 02313), with the upper part showing thewahgene model, the two neighbouring editing sites (indicated by the red arrow below the 9th exon) and their recoding potential. The two black vertical arrows above the gene model indicate the exon regions that code for the PEHE domain. The histograms show the editing levels of the editing sites in the nine head samples.P-values of Fisher’s exact tests between any two of the three castes within the same colony are given above the bars (*P<0.05, **P<0.01, ***P<0.001.P-values between 0.05 and 0.1 are given in precise figures). 2d,e , Supplementary Table 5 and Supplementary Methods ) with around half located within 20-bp of neighbouring editing sites ( Supplementary Fig. 3d ). To further confirm the accuracy of our methods and data sets, we randomly selected 116 editing sites, including 106 A-to-I editing sites and 10 non-A-to-I editing sites, for experimental validation using PCR amplification, TA cloning and Sanger sequencing (see Methods). Overall, 110 of these 116 sites (95%) were confirmed, but validation percentages differed between A-to-I editing sites (99%; 105/106) and non-A-to-I editing sites (50%; 5/10) ( Supplementary Data 1 ). As non-A-to-I editing is rare and apparently more difficult to validate, we decided to use only the A-to-I editing sites in further analyses. Our PCR and cloning validations further showed that the editing levels calculated by our initial pipeline were consistent with the levels obtained by TA-clonal sequencing (Pearson’s r =0.76 and P <10 −15 for all 116 editing sites; Pearson’s r =0.78 and P <10 −15 for the 106 A-to-I sites; Supplementary Fig. 4 ). On average, ca . 42% of the A-to-I editing sites targeted genic regions, particularly the 3′-untranslated regions (3′-UTRs) (obs./exp.=21%/7%), whereas protein-coding regions (coding sequences (CDSs)) tended to be depleted of RNA-editing sites (obs./exp.=1%/19%) ( Fig. 2c ). Similar depletion of A-to-I editing sites in CDSs has been documented in humans [17] , mice [16] and C. elegans [13] , but fruit flies have substantial enrichment of A-to-I editing sites in their CDSs (28% of total, data from ref. 15 ). Our results for a fungus-growing ant thus imply that enrichment of CDS RNA editing in Drosophila may be the exception rather than the rule for insects. However, 77% of the CDS-editing sites in A. echinatior had the potential to change protein sequences, mainly by recoding amino acids ( ca . 99%), but in a few cases by removing stop codons ( Supplementary Table 6 ). In addition, CDS-editing sites were less likely to be clustered compared with editing sites in other genomic elements ( Fig. 2d ), which is unlikely to be simply due to the low number of CDS-editing sites, as 5′-UTRs harbour similarly low numbers ( Fig. 2c ). We also found that simultaneous editing of genes in UTRs, CDSs and introns was rare, and that only a few genes were in fact edited in more than one of these genic regions ( Fig. 2f ). Up to 32% of A-to-I editing sites occurred in transposable elements (TEs), a figure that was four times higher than the background expectation of 8% ( Fig. 2c ). The fact that TE transcripts are another major target of RNA editing in A. echinatior is interesting, because only one case of RNA editing in TE transcripts has been reported in insects: A-to-I, U-to-C and C-to-U editing in read-through transcripts of the KP elements of Drosophila melanogaster [35] . In humans, A-to-I editing is pervasive in Alu repeats [19] , a primate-specific short interspersed element that represents about 10% of the entire human genome [37] . Our data thus provide the first evidence for substantial RNA editing in insect TEs, and may imply that the activity of a significant fraction of A. echinatior TEs is regulated by RNA editing. Functional editing sites shared across colonies Comparing the A-to-I editing sites among samples of the same caste from different colonies, we found that ca . 60% (range 43–76%) of the caste-specific editing sites were shared by the three sampled colonies ( Fig. 3a–c ). This indicates a marked disparity of RNA-editing events among sympatric colonies of the same species, consistent with the limited reproducibility of editing events among different human individuals [17] , [20] . This variability may be due to colony-specific habitat conditions, colony size, colony age or even random expression noise. However, as our focus was on the editing sites most likely to contribute to caste-specific functions, we continued our analyses using only those sites where editing was confirmed in samples of a caste across all three colonies. This allowed us to identify 4,682, 5,049 and 9,120 caste-specific A-to-I editing sites for gynes, large workers and small workers, respectively ( Fig. 3a–c ), representing a total of 10,282 sites that were consistently edited in at least one caste. The high number of small worker-specific editing sites could not be explained by variation in sequencing depth among samples ( Supplementary Fig. 5 ), but corresponded with the higher expression level of ADAR in small workers ( Fig. 1c ). Figure 3: Functional editing sites in the leaf-cutting ant A. echinatior . ( a – c ) Venn diagrams of A-to-I editing sites across the three different colonies Ae322, Ae356 and Ae363. ( d ) Over-represented Gene Ontology (GO) terms for the 835 genes that were consistently edited in at least one caste, showing the percentages of edited genes relative to all transcribed genes annotated to corresponding GO terms. The first number after each bar indicates the number of edited genes annotated to this GO term, and the second number indicates the number of all transcribed genes (RPKM >1 in at least one of the nine sequenced samples) annotated to this GO term. Full size image We identified 533, 538 and 779 genes that harboured at least one consistently edited site in gynes, large workers and small workers, respectively, corresponding to a total of 835 genes ( Supplementary Data 2 ). The most highly edited gene was Aech_13462 , with >70 consistently edited sites in its 3′-UTR in all three castes ( Fig. 2e and Supplementary Data 2 ). This gene is an orthologue of Mdh1 (malate dehydrogenase 1), which has a conserved role in aerobic energy production [38] . The high expression level of this gene in the heads of Acromyrmex leaf-cutting ants (mean RPKM (reads per kilobase of transcript per million reads mapped) across 9 samples: 264; Supplementary Methods ) probably implies that the aerobic energy requirements for brain activity are extremely high, and extensive RNA editing of its 3′-UTR may reflect a continuous need for fine-tuning gene expression related to energy metabolism. Another gene with a considerable number of consistently edited sites was Aech_00116 , an orthologue of Hsc70-4 (heat shock 70-kDa protein cognate 4) in Drosophila , which is involved in nerve-evoked neurotransmitter exocytosis, a process critical for signal transmission across synapses [39] . It had >50 consistently edited sites in its 3′-UTR in all 3 castes of A. echinatior ( Supplementary Data 2 ), which may offer a special mechanism for post-transcriptional regulation of this gene. Gene Ontology (GO) enrichment analysis for the 835 genes, which were consistently edited in at least 1 caste (using all expressed genes as background), showed that 5 functional categories were over-represented among the RNA-edited genes, including neurotransmission, circadian rhythm, response to temperature stimulus, RNA splicing and carboxylic acid biosynthesis ( Fig. 3d ; see Methods). Functions in neurotransmission, including GO terms of synaptic growth at neuromuscular junctions, synaptic transmission and cell signalling, are consistent with the known functions of RNA editing in animal nervous systems [10] . For example, we found RNA editing in a series of genes encoding voltage-gated ion channel proteins, such as Shab (K + channel), Shaw (K + channel), Hk (K + channel), NaCP60E (Na + channel) and Ca-alpha1T (Ca + channel), as well as some neurotransmitter secretion-related proteins, such as Snap25 (Synapse protein 25), n-syb (n-synaptobrevin), Sytbeta (Synaptotagmin beta) and Syt12 (Synaptotagmin 12) ( Supplementary Data 2 ). Circadian rhythms have rarely been reported to be affected by RNA editing, although the previous discovery of RNA editing of the qvr and Sh transcripts in Drosophila is consistent with this possibility [40] . Yet, in A. echinatior we observed editing of many circadian rhythm genes: including qvr (quiver) [41] , Shaw (Shaker cognate w) [42] , lark [43] , nocte (no circadian temperature entrainment) [44] , Atf-2 (Activating transcription factor-2) [45] , cyc (cycle) [46] , ctrip (circadian trip) [47] , CkIIα (casein kinase IIα) [48] and Rdl (Resistant to dieldrin) [49] ( Supplementary Data 2 ). Extensive RNA editing of circadian rhythm genes suggest that ants may possess a novel mechanism for adjusting circadian sleep/wake cycles with very short response times. We only identified 27, 38 and 53 CDS-editing sites with amino acid recoding potential that were consistently edited in gynes, large workers and small workers, repectively, representing a total of 57 sites targeting 34 genes ( Supplementary Data 3 ). Thirty-three per cent (19/57) of these recoding sites were located within or near (within 20 amino acids) known protein domains ( Supplementary Data 3 ). The majority of these recoded genes were implicated in neural system functions such as synaptic transmission (for example, Caps and qvr ), neurogenesis (for example, ctrip and Ars2 ), neuromuscular junction development (for example, TBPH and wah ) and circadian rhythm (for example, qvr and ctrip ). There were also some genes involved in mitotic processes (for example, RpL7 and Mtor ), RNA splicing (for example, CG7564 and CG2926 ) and organism development (for example, rhea and scra ) ( Supplementary Data 3 ). Conservation of RNA editing in ants RNA editing may be conserved at two levels: the conservation of genomic sites corresponding to RNA-editing sites (DNA level) and the conservation of the RNA-editing events themselves (RNA level). We recently sequenced and assembled the genomes of another five attine fungus-growing ant species (Nygaard et al. , in preparation) which, together with the published genomes of A. echinatior [32] and Atta cephalotes [50] , span the most recent ca . 25 MY of the attine ant lineage that originated ca . 50 MYA [30] . Combining these data with the published genomes and transcriptomes of two non-fungus-growing ants, C. floridanus (Florida carpenter ant) and H. saltator (Jerdon’s jumping ant) that diverged from A. echinatior ca . 80 and 100 MYA [8] , [51] , [52] , we had the opportunity to estimate the degree of conservation of RNA editing in ants over long evolutionary time scales. Whole-genome alignment analysis (see Methods) showed that 67% of all transcribed ‘A’s (that is, ‘A’s covered by more than a single RNA read in at least one caste) in A. echinatior were highly conserved (that is, displaying the same DNA base) among the 7 attine ant species, while 57% and 46% were conserved when comparing A. echinatior with C. floridanus and H. saltator , respectively. However, when we assessed the editing sites that appeared in at least one caste across all three colonies, we found that only 23% of these RNA-editing sites were conserved across the seven attine genomes and about 11% and 8% between A. echinatior and C. floridanus or H. saltator , respectively. The latter conservation percentages were all significantly lower than the former genome background percentages (Monte Carlo test P <10 −4 ). Similar patterns were observed when we extended these comparisons to the separate genomic elements ( Fig. 4a , Supplementary Fig. 6 and Supplementary Table 7 ). Figure 4: Conservation of RNA editing among ant species. ( a ) Percentage of conserved genomic sites that display the same DNA bases among seven attine ant species. The ‘Gene’ category is the sum of 5′-UTRs, 3′-UTRs, CDSs and introns, and the ‘Intergenic’ category represents all genomic regions that are neither genes nor TEs. The red bars (genome background) were calculated from all transcribed ‘A’s (that is, ‘A’s covered by ≥1 RNA reads) in each category, and the blue bars from genomic sites corresponding to A-to-I RNA editing sites in each category. ( b ) The number of conserved editing events (sites displaying the same RNA base substitutions among species) between A. echinatior and C. floridanus and between A. echinatior and H. saltator . ( c ) Correlation of RNA-editing levels for the conserved editing events between heads of small workers of A. echinatior and brains of minor workers of C. floridanus . Only sites with RNA read coverage ≥10 × in both samples were used. Editing levels of A. echinatior small workers were calculated from the combined data of the three small worker samples. The blue line is a linear regression that is virtually identical to the diagonal. ( d ) Editing of the qvr gene in A. echinatior . The upper part shows the qvr gene model and the two editing sites, as well as their protein recoding potential. The red arrow in the sixth exon indicates the positions of the two neighbouring editing sites. The lower part shows the editing levels of the two sites in the nine head samples (G, L, S stand for gynes, large workers and small workers, respectively, and are followed by colony number). ( e , f ) Editing levels of the corresponding sites of qvr in C. floridanus and H. saltator . Full size image We also estimated the conservation status of the genomic sites with RNA editing by using phastCon scores (base-by-base conservation scores ranging from 0 to 1) derived from the multiple genome alignments for the seven attine ant species (see Methods), and observed that the mean phastCon scores of genomic sites corresponding to RNA-editing sites were significantly lower than those of random genomic sites ( Supplementary Table 8 ). Taken together, these results suggest that genomic sites with RNA editing are fast evolving, and imply that most RNA-editing sites in A. echinatior are species-specific and thus likely to have emerged recently. To further investigate why genomic sites corresponding to RNA-editing sites appear to evolve relatively fast, we checked the evolutionary rate of the 835 genes, which contained at least 1 caste-specific editing site that consistently appeared in 3 colonies by calculating the non-synonymous ( dn ) and synonymous ( ds ) mutation rate among the 7 attine ant species ( Supplementary Methods ). Except for the small proportion of 5′-UTR-edited genes, we generally found that the coding regions of RNA-edited genes evolved at equal or lower rates than the background genes ( Supplementary Fig. 7 ). This suggests that the fast evolutionary rate of RNA-editing sites cannot be explained by hitchhiking effects connected to neighbouring genes. It thus seems more probably that the fast evolution of RNA-editing sites may relate to gene expression responses to changes in the specific social environments of different fungus-growing ant species. We next examined whether RNA editing of the conserved A. echinatior genomic sites also occurred in the transcriptomes of other ant species by comparing the RNA editomes of A. echinatior with previously published transcriptome data from C. floridanus and H. saltator ( Supplementary Table 9 ) [8] , [9] , [51] . We identified 113 and 84 A. echinatior sites that were also edited and displayed the same RNA base substitutions in at least one sample of C. floridanus and H. saltator , respectively. We identified 45 sites that displayed the same RNA base substitutions in all three ant species ( Fig. 4b ). The number of conserved RNA-editing events that this analysis identified is likely to be an underestimate because the transcriptome sequencing depth in C. floridanus and H. saltator was lower than in A. echinatior , and samples were obtained in different ways [8] , [9] , [51] . Yet, 33 of the 45 sites (73%) with conserved editing events were targeting 20 genes of A. echinatior and 18 of these sites were edited in protein coding regions with amino acid recoding potential ( Supplementary Data 4 ). Functional analysis based on orthologues in Drosophila revealed that 8 of the 20 A. echinatior genes with conserved editing (40%) were involved in neural activity or circadian rhythm. For example, qvr (also called sleepless ), a gene participating in the regulation of circadian sleep/awake cycles in Drosophila [41] , harbours two A-to-I editing sites in the last exon in all three castes of A. echinatior and in most samples of C. floridanus and H. saltator , causing S101G and H106R amino acid recoding in the protein sequence ( Fig. 4d–f ). Multiple sequence alignments indicated that genomic sites corresponding to these two editing sites are highly conserved in many insect species ( Supplementary Fig. 8 ). Surprisingly, the qvr A-to-I RNA editing that we discovered occurs on exactly the same two sites in Drosophila [40] , indicating that both editing events have been conserved for >300 MY of insect evolution. Other examples include the following: Rdl and lark , two genes involved in circadian rhythm [43] , [49] ; TBPH (also called TDP-43 ), a gene associated with neuromuscular junction development [53] ; Caps (calcium-activated protein for secretion), a gene involved in synaptic transmission [54] ; and tipE (temperature-induced paralytic E), a gene encoding voltage-gated sodium channel auxiliary subunits ( Supplementary Data 4 ). These results once more confirm the importance of RNA editing in the regulation of nervous system function in A. echinatior . Finally, the conserved editing events between head samples of A. echinatior and brain samples of C. floridanus allowed us to estimate the correlation of editing levels in similar tissues between the two ant species. We found that editing levels in A. echinatior were positively correlated with editing levels in C. floridanus at the same sites ( Fig. 4c,e,f ), implying that not only the editing events but also the degrees of editing have probably been under similar selection for many of these sites. RNA editing and behavioural caste differentiation In general, we observed that genome-wide editing patterns were quite similar across samples of the same caste from different colonies, with hierarchical clustering analysis separating samples by caste ( Fig. 5a ), which indicates that RNA-editing profiles differ more across castes than across colonies. Moreover, consistent with the ADAR expression pattern across the three castes ( Fig. 1c ), RNA-editing patterns of large workers were closer to those of gynes than small workers ( Fig. 5a ). Figure 5: Caste-specific RNA editing in A. echinatior . ( a ) Heatmap and hierarchical clustering based on editing levels of all the editing sites identified in the nine samples (G, L, S stand for gynes, large workers and small workers, respectively, and are followed by colony number). Sites for which editing was confirmed in at least one of the nine samples and that had RNA read depth ≥20 × in all the nine samples were used ( n =2,944). ( b ) Percentages of the 137 consistently differentially edited sites across different genomic elements. The ‘Gene’ category is the sum of 5′-UTRs, 3′-UTRs, CDSs and introns, and the ‘Intergenic’ category represents all genomic regions that are neither genes nor TEs. ( c ) RNA editing of wah (Aech 02313), with the upper part showing the wah gene model, the two neighbouring editing sites (indicated by the red arrow below the 9th exon) and their recoding potential. The two black vertical arrows above the gene model indicate the exon regions that code for the PEHE domain. The histograms show the editing levels of the editing sites in the nine head samples. P -values of Fisher’s exact tests between any two of the three castes within the same colony are given above the bars (* P <0.05, ** P <0.01, *** P <0.001. P -values between 0.05 and 0.1 are given in precise figures). Full size image We used Fisher’s exact tests to identify sites that displayed significantly different levels of RNA editing between any two of the three female castes within each colony (see Methods) and detected an average of 276, 599 and 338 significantly differentially edited sites between gynes/large workers, gynes/small workers and large/small workers, respectively ( Supplementary Table 10 ). To focus on sites where editing changes are likely to be persistently associated with caste status rather than colony age, colony size or habitat, we restricted our further analyses to target differentially edited sites that were shared across the three sampled colonies (see Methods) and identified 10, 124 and 15 sites with consistently different editing levels across the three colonies for gyne/large worker, gyne/small worker and large/small worker comparisons, respectively, which involved a total of 137 sites targeting 48 genes. Of these 137 consistently caste-differentially edited sites, 43, 13 and 13 were conserved for their corresponding genomic sites among the 7 attine ants, between A. echinatior and C. floridanus , and between A. echinatior and H. saltator , respectively. This encompassed a total of 55 sites, representing 40% of the 137 differentially edited sites ( Supplementary Data 5 ). Three of these sites were located in protein coding regions, with two of them targeting the ninth exon of the gene Aech_02313 , which had significantly higher editing levels across colonies in small workers compared with gynes, and resulted in Q966R and Q968R amino acid recoding in the protein sequences ( Fig. 5c ). This gene is an orthologue of the wah gene (also known as NSL1 , CG4699) in D. melanogaster and has been proposed to participate in neuromuscular junction development [55] . We found that editing of these two sites was always linked ( Supplementary Table 11 ), and domain annotation revealed that they were close to the PEHE domain (histone acetyltransferase binding activity) of the wah gene ( Fig. 5c ), implying their potential to affect protein activity. Both of these two recoding sites were highly conserved in ants ( Supplementary Fig. 9a,b ) and Q968R was also edited in some samples of C. floridanus and H. saltator ( Supplementary Fig. 9c ). Another site in which small workers showed significantly higher editing levels than gynes across colonies, was targeting the fifth exon of Aech_08485 : a gene encoding a Zinc finger protein ( Supplementary Fig. 10 ). This editing site can cause K432R recoding in the protein sequence downstream of the C2H2 zinc finger domain and is also conserved in all other ant species and edited in some samples of C. floridanus ( Supplementary Fig. 11 ), but no function for this gene is known. Most of the consistently differentially edited sites were targeting the non-coding regions of genes, mainly in 3′-UTRs ( Fig. 5b ), some of which are known to function in neural systems ( Supplementary Data 5 ). For example, Tap42 , pUf68 and Droj2 are known to participate in neurogenesis in Drosophila [56] , and all of them harboured consistently differentially edited sites in their 3′-UTRs that displayed higher editing levels in worker castes than in gynes ( Supplementary Fig. 12 and Supplementary Data 6 ). Another gene associated with neuromuscular junction development, TBPH (also called TDP-43 ) [53] , also harboured a consistently differentially edited site in its 3′-UTR with higher editing levels in small workers than in gynes ( Supplementary Fig. 12 and Supplementary Data 6 ). The neuromuscular junction connects the nervous system to the muscular system via synapses between nerves and muscle fibres, and is critical in locomotory behaviour. Differential editing of TBPH and wah may thus imply that RNA editing is involved in modulating caste-specific adult locomotory behaviour. RNA editing in the 3′-UTR of genes cannot change protein sequences, but may affect the stability of mRNA or change the targets of miRNAs [25] to regulate the final protein levels. Moreover, it has been proposed that A-to-I RNA editing may cross-talk with RNA-interference pathways, which involve dsRNAs; thus, RNA editing may play a role in gene silencing (reviewed in ref. 57 ). The differential patterns of RNA editing among A. echinatior castes thus appear to uncover a suite of novel potential mechanisms for differentiating caste phenotypes in eusocial insects. This is the first study focusing on the characteristics and functions of RNA editing in a eusocial insect. Unlike previous studies, we used a strand-specific RNA-Seq strategy, which can infer editing types directly from the sequencing reads, independent of whether genomic annotations are available. Our study also exploited the fact that A. echinatior , similar to most other eusocial Hymenoptera, has low degrees of genetic polymorphism within single colonies (our sampling unit) because all females are offspring of the same (diploid) mother queen and four to eight haploid males [58] . Our high-coverage sequencing for gDNA and RNA thus allowed us to capture essentially all genetic variation present in these colonies. We acknowledge that some of the low-level RNA editing events could represent false positives due to errors in the amplification or sequencing processes, but also note that scatter for low editing level estimates obtained with two independent methods was low; hence, this is unlikely to affect our main conclusions ( Supplementary Fig. 4 ). Consistent with observations in other animals, A-to-I editing appeared to be the dominant form in ants, with >96% of the identified editing sites belonging to this category, supporting the view that non-A-to-I RNA editing is very rare in animals. The highly similar characteristics of A-to-I editing sites among ants, humans, mice and fruit flies, such as their frequent occurrence in clusters and in dsRNA regions, and their analogous depletion/enrichment of guanines in the upstream/downstream positions of edited adenosine, strongly suggest that the function of ADAR enzymes is highly conserved from insects to mammals, regardless of the variation in copy numbers of ADAR genes across lineages. In addition, two novel characteristics of RNA editing were reported in this study: (i) the low clustering tendency for editing in coding regions compared with editing in other regions and (ii) the mutually exclusive editing of different regions within gene bodies. Our finding of RNA-edited genes that are functionally enriched for neurotransmission and circadian rhythm is consistent with the known role of RNA editing in the nervous systems, but also offers extensions to the spectrum of possible functions of RNA editing. Our results suggest a new and potentially wide-ranging post-transcriptional gene regulation mechanism that could fine-tune gene expression in the eusocial insect brain. Eusocial insects, such as ants, combine individual and collective behaviours in a uniquely self-organized manner [59] , which might be particularly amenable to regulatory mechanisms such as RNA editing. However, much further work will be needed to detail the relative importance of alternative mechanisms that determine the expression of genes affecting ant behaviour. Comparative analyses among both closely and distantly related ant species revealed mostly low levels of conservation in the genomic sites whose transcripts are subject to RNA editing, suggesting that most editing sites may have emerged in the recent history of A. echinatior . However, other genomic regions, representing 8–23% of the RNA-editing sites, appear not to have changed for hundreds of millions of years, indicating they have been under purifying selection during the very long evolutionary history of the ants since their single ancestor became eusocial [60] . The regulatory functions of RNA editing at the latter sites may hold important information about the fundamental origins of eusocial organization to be uncovered in future studies. In addition, the cross-species conservation of the relatively small number of RNA-editing sites that showed consistently different editing levels across adult caste phenotypes may offer valuable insights into the mechanisms that made eusociality in ants progress almost immediately towards morphological caste differentiation with distinct behavioural syndromes. In eusocial lineages of bees, wasps and termites, initial caste differentiation appears to have been based on conditionally expressed, reversible behaviours that did not become associated with permanent morphological castes until much later in their evolutionary history [61] , [62] , [63] , [64] . Analysis of RNA editing enzymes We obtained ADAR protein sequences of Apis mellifera (NP_001091684.1), D. melanogaster (NP_569940.2), C. elegans (NP_492153.2, NP_498594.1), N. vectensis (XP_001642062.1, XP_001629615.1), C. gigas (EKC20855.1, EKC32699.1) and C. intestinalis (XP_002122509.2, XP_002128212.1) from NCBI, Homo sapiens (ENSP00000292205, ENSP00000435381, ENSP00000370713) and Xenopus tropicalis (ENSXETP00000008359, ENSXETP00000057325, ENSXETP00000039188) from Ensembl (release-68), and S. purpuratus (SPU_008095, SPU_012470) from EnsemblMetazoa (release-18), and used these sequences as queries to search for ADAR genes in seven published ant genomes ( http://hymenopteragenome.org/ant_genomes/ ) and five unpublished ones (S. Nygaard et al. , in preparation). We first mapped the query proteins to the ant genomes with TBLASTN (v2.2.23) and excised target-gene regions (2-kb flanking sequences) for gene structure and protein sequence determination using GeneWise (v2-2-0). Next, we aligned the predicted proteins to the nr database of NCBI to check whether the predicted proteins were ADARs. The gene model in Solenopsis invicta was only partially assembled and omitted from further analysis. Domain organization of the ADAR proteins was then predicted using Pfam ( http://pfam.sanger.ac.uk ) with default settings. Conservation scores of the ADAR proteins among the 11 ant species were analysed in http://compbio.cs.princeton.edu/conservation/ , which uses the Jensen–Shannon divergence to quantify the conservation level [65] . Phylogenetic analysis was performed using MEGA5 ( http://www.megasoftware.net ). To search for APOBEC genes in the insect genomes, we collected the APOBEC protein sequences of H. sapiens (APOBEC1, APOBEC2, APOBEC3A-3H and APOBEC4), X. tropicalis (apobec2 and apobec4) and Danio rerio (apobec2a and apobec2b) from Enesmbl (release-68) and performed the same analysis as described above. No homologues could be identified in any of the 12 ant genomes and other insects with available genomes. Biological material and DNA/RNA extraction Three colonies of A. echinatior (Ae322, Ae356 and Ae363) were collected in Gamboa, Panama, in 2006–2008, and maintained in the laboratory under standard conditions of ca . 25 °C and ca . 70% relative humidity where they were supplied with a diet of bramble leaves, rice and pieces of apple. RNA and DNA samples were collected from the three female castes: gynes, large workers and small workers. Animals were flash frozen in liquid nitrogen and the heads separated from the bodies with a pair of forceps. Heads from 50 gynes, 50 large workers or 200 small workers originating from the same colony were pooled and used for RNA extraction as described previously [66] . The remaining body parts were likewise pooled per caste and colony, and subsequently used for DNA extraction ( Supplementary Table 1 ). gDNA was extracted using a Blood & Cell Culture Midi kit (Qiagen) following the manufacturer’s instructions, with the modification that sample lysis was performed overnight. qPCR analysis of ADAR and GADPH expression Total RNA of the nine samples was first converted to complementary DNA using SuperScript II reverse transcriptase (Invitrogen) and an oligo d(T) primer according to the manufacturer’s instructions. Forward and reverse primers for ADAR were 5′-GCT GAC CAA ATT GGC AAG AT-3′ and 5′-CCG CTT CGA CTT AAA TGC TC-3′, respectively, and forward and reverse primers for GADPH were 5′-AGC CAC TCA GAA GAC CGT TG-3′ and 5′-CCA GTA AGC TTC CCG TTG AG-3′, respectively. Primer pairs were spanning an intron to prevent amplification of gDNA. The final PCR reactions contained 0.8 μl of each primer (10 μM), 10 μl SYBR Green I (TaKaRa) and 2 μl template. Quantitative PCR (qPCR) was performed on an ABI StepOnePlus System using Ex Taq HS polymerase (TaKaRa) in a final volume of 20 μl and the Ef1-beta gene (primers: 5′-CCA CAG TTA TTG CCA AAT CG-3′ and 5′-ACC CAC TGG GAC AAG TTT TG-3′) as internal reference. All reactions were subjected to 95 °C for 10 min followed by 40 cycles of 95 °C for 15 s and 60 °C for 1 min, and melting curve analysis to ensure homogeneity of the reaction product. qPCR results were analysed using the StepOne Software. Library construction and sequencing For each DNA sample, 5 μg gDNA was fragmented by sonication with a Covaris S2 system (Covaris, MA) to a mean size of ~500 bp, followed by end repair, 3′-end addition of dATP and adapter ligation. The ligated fragments were size selected at 500 bp on an agarose gel and amplified by ten cycles of PCR to yield the DNA libraries. All libraries were subjected to 90 bp paired-end sequencing on an Illumina HiSeq 2000 platform. Strand-specific RNA-Seq libraries were constructed according to Parkhomchuk et al. [36] Briefly, 2 μg total RNA per sample was treated with DNase I (New England BioLabs) to remove possible contamination with gDNA. Next, poly (A+) mRNA was purified from the total RNA using the Dynabeads mRNA Purification Kit (Invitrogen), followed by fragmentation using the RNA fragmentation kit (Ambion). Next, the first cDNA strand was synthesized using random hexamer primers and reverse transcriptase (Invitrogen), and second-strand cDNA was synthesized using DNA polymerase I (New England BioLabs) where dUTP was used instead of dTTP. After that, the synthetic double-stranded cDNA was end repaired, followed by 3′-end addition of dATP, adapter ligation and size selection according to Illumina’s protocols. Finally, the selected products were treated by UNG (Applied Biosystems) and amplified by 15 cycles of PCR to yield the strand-specific RNA-Seq libraries. All the libraries were subjected to 90 bp pair-end sequencing on the Illumina HiSeq 2000 platform. Read alignment RNA and DNA reads were aligned to the genome of A. echinatior [32] (Aech_2.0_scaffolds.fa.gz from http://hymenopteragenome.org/acromyrmex/ ) using BWA (v0.5.9-r16), allowing five mismatches and zero gaps for the 90-bp reads. Only uniquely mapped reads (XT:A:U) with mapping quality ≥20 and with no suboptimal hits found by BWA (X0:i:1 and X1:i:0) were kept for further analysis. Reads resulting from PCR duplications (that is, read pairs that mapped to identical genomic locations) were removed except for the one with the highest sequencing quality. We then cut the first and last 6-bp of the aligned reads, as it is known that (i) the error rate of Illumina sequencing is higher towards both ends of a read, especially at the 3′-end; (ii) some 5′-end mismatches may be introduced by the random hexamers during the first- and second-strand syntheses of RNA library construction; and (iii) mapping errors around insertions/deletions relative to a reference genome can lead to mismatches occurring towards the beginning and ends of a read. In addition, to improve the accuracy of read alignment, we used BLAT (v. 34) to re-align all the uniquely mapped reads to the reference genome and only kept reads supported by both BLAT and BWA. As the fundamental algorithms of BLAT and short-read aligners such as BWA are different, the read-mapping results were often different and complementary, especially in handling reads derived from spliced junctions [18] . Finally, ca . 63% of the raw DNA data and ca . 29% of the raw RNA data were retained for further analysis ( Supplementary Table 2 ). Identification of RNA-editing sites The basic principle for identifying an RNA-editing site is that the site must be homozygous for gDNA, while at the same time displaying a mismatch between RNA and DNA. We conducted two rounds of editing site identification in each sample. In the first round, we required that (i) a candidate RNA-editing site in a given sample must be supported by ≥3 RNA reads that were mapped to overlapping but not identical positions in the reference genome and this site had an editing level ≥5%. The editing level of a candidate editing site was calculated as the number of reads supporting editing divided by the total number of reads covering that site. RNA reads with quality score <30 for the candidate editing positions were discarded (that is, the upper limit of sequencing error for a base was 0.1%). (ii) The candidate sites with multiple editing types were discarded. (iii) To avoid potential false positives resulting from mis-mapping of reads at splice junctions, we further required a candidate editing site to be supported by at least one RNA read in the middle of its length (that is, from positions 23–68 of the 90-bp read), and we discarded intronic candidate sites that occurred within 10 bases of an splice site. (iv) To remove false positives resulting from heterozygous genomic SNPs, we only kept candidate editing sites in homozygous genomic sites. Taking into account that female offspring are most likely to be half-sisters because queens of A. echinatior mate with multiple males [58] and that our samples were pools of multiple individuals, some heterozygous alleles may have occurred in low frequencies in our data set, making commonly used SNP calling algorithms unsuitable as tools. Thus, to filter as many heterozygous SNPs as possible, we defined homozygous genomic sites with a strict criterion: sites with ≥10 × DNA read coverage in each of the 9 samples and all the covering reads supporting the same genotype in all the 9 samples. DNA reads with quality score <30 for the interrogated positions were discarded. (v) Finally, to avoid potential false positives resulting from mis-mapping of reads between very similar paralogous regions, we removed candidate editing sites in regions that were >90% similar to other parts of the genome based on a self-to-self whole-genome alignment using LASTZ (v1.01.50; http://www.bx.psu.edu/miller_lab/ ), and we discarded candidate editing sites with DNA reads depth of more than twice the genome-wide peak depth in any of the nine samples. As most editing sites have very low editing levels ( Fig. 2b ) and some also had low coverage, a number of true-positive editing sites may have been missed due to the stringent filtering criteria outlined above. To retrieve such missed editing sites, we conducted a second round of editing-site identifications. We first combined all editing sites identified in the first round to obtain a comprehensive map of potentially editable positions in the genome of A. echinatior , which produced a total of 17,229 positions that were confirmed to be homozygous for gDNA, to be located in unique genomic regions, to not be close to any splice sites and to be edited in at least one of the 9 samples. We then retrieved missed editing sites in each sample using the more liberal criterion of sites with ≥1 RNA read, supporting editing in already identified editable positions also being permissible. To further distinguish between true and false positives due to sequencing error, we performed statistical tests for the candidate editing sites identified in each sample based on the binomial distribution B( n , p ), with p =0.1% (the upper limit of sequencing error for a base required in this study) and n equal to the total depth of a candidate editing site. For example, given a candidate editing site with k reads supporting editing and a total depth of n , we calculated the probability that all the k reads sequenced in the n trials were false positives at a specific candidate editing position, and then compared the probability of B( k , n , p ) to 0.01 after adjusting the P -value by Benjamini–Hochberg False discovery rates (FDRs) [67] . Only candidate editing sites with adjusted P -values <0.01 were finally considered to be true positives and kept for subsequent analyses. PCR validation of identified RNA-editing sites To confirm the reliability of our pipeline, we randomly picked 116 editing sites from large workers of colony 363 (L363) for PCR validation, including 106 A-to-I editing sites and 10 non-A-to-I editing sites that were distributed in 21 PCR amplicons. The gDNA and RNA samples of L363 used for PCR validation were the same as the ones used in the DNA- and RNA-Seq experiment described above. Total RNA was first converted to cDNA using SuperScript II reverse transcriptase (Invitrogen) with oligo d(T) according to the manufacturer’s instructions. Next, for each site we amplified a fragment spanning the editing site from both the gDNA and the cDNA samples (primers listed in Supplementary Data 1 ). PCR products from gDNA samples were subjected to Sanger sequencing on an ABI 3730 DNA sequencer, and PCR products from cDNA samples were used to construct TA clones of which we randomly selected ca . 50 for Sanger sequencing on the same ABI 3730 sequencer to validate the existence of RNA editing. An editing site was considered to be true when its gDNA was homozygous based on the .ab1 chromatogram file and at least 1 out of the 50 sequenced clones supported editing. The editing level for each editing site was subsequently calculated as the number of clones with the edited nucleotide divided by the total number of sequenced clones. Functional annotation and enrichment analysis GO annotations for A. echinatior genes were based on orthologues in C. elegans , D. melanogaster , A. mellifera , Nasonia vitripennis and A. cephalotes from EnsemblMetazoa (release-18). Fisher’s exact test and χ 2 -test were employed to estimate whether a list of edited genes was enriched in a specific GO category when compared with background genes [68] . All expressed genes, which we defined as genes with RPKM >1 in at least one of the nine sequenced samples, were used as background genes in this GO enrichment analysis. P -values were adjusted for multiple testing by applying FDR [67] . Conservation analysis of RNA-editing sites To investigate the evolutionary conservation of genomic sites corresponding to RNA-editing sites, we performed cross-species whole-genome alignments between A. echinatior and six other attine ants ( A. cephalotes , Atta colombica , Trachymyrmex septentrionalis , Trachymyrmex cornetzi , Trachymyrmex zeteki and Cyphomyrmex costatus ) plus two non-attine ants ( C. floridanus and H. saltator ). Whole-genome alignments were performed using LASTZ with default parameters and using the A. echinatior genome as the reference. Two methods were used to estimate the conservation degrees of the genomic sites corresponding to RNA-editing sites: (i) the percentage of genomic sites corresponding to RNA-editing sites showing the same DNA bases among seven attine ant species, between A. echinatior and C. floridanus and between A. echinatior and H. saltator , respectively; and (ii) mean phastCons scores for genomic sites corresponding to RNA-editing sites, which were calculated from the multiple genome alignments of the seven attine ant species. For both methods, Monte Carlo simulations were performed to estimate whether the observed conservation degrees were significantly different from that of background expectation. Briefly, the same number of transcribed ‘A’s (RNA read coverage ≥1 × ) as that of A-to-I editing sites was randomly sampled in each genomic element, then the conservation degrees for each element were calculated. The p -value for each element was empirically calculated after the simulation of 10,000 iterations, and the expected conservation degree was the mean value of the 10,000 iterations ( Supplementary Tables 7 and 8 ). To identify conserved editing sites, we performed cross-species transcriptome comparisons between A. echinatior and C. floridanus (or H. saltator ). RNA-Seq data of different developmental stages and castes of C. floridanus and H. saltator were collected from three studies [8] , [9] , [51] ( Supplementary Table 9 ) and whole-genome BS-Seq data from Bonasio et al. [8] (GSE31576 in NCBI GEO database) were used for removing potential heterozygous SNPs. A conserved editing site between A. echinatior and C. floridanus (or H. saltator ) was defined as a homozygous genomic site with consistent genotype and consistent editing type between A. echinatior and C. floridanus (or H. saltator ). Considering the generally lower sequencing depth of the RNA-Seq samples of C. floridanus and H. saltator , we required a conserved editing site to be supported by ≥1 RNA reads in at least one of the C. floridanus (or H. saltator ) samples. Hierarchical clustering analysis for RNA-editing sites All editing sites that were confirmed in at least one of the nine sequenced samples by our pipeline and that had RNA read depth ≥20 × in all the nine samples were used for hierarchical clustering analysis ( Fig. 5a ). The method for distance measurement was ‘euclidean’ and the agglomeration method was ‘complete’. The heatmap as well as the hierarchical clustering tree were generated by the pheatmap function in R ( www.r-project.org ) based on the editing levels of the editing sites. Identifying sites with caste-specific RNA editing For the analysis of differential editing, we first identified differentially edited sites between any two castes within each individual colony (giving nine comparisons in total). To ensure that difference in editing levels between two castes were not due to random variation or insufficient coverage depth in one of the two samples, we performed Fisher’s exact test for each interrogated site. The four variables subjected to Fisher’s exact test for each site were (i) the number of RNA reads supporting editing in caste one, (ii) the number of RNA reads supporting non-editing in caste one, (iii) the number of RNA reads supporting editing in caste two and (iv) the number of RNA reads supporting non-editing in caste two. Only sites with P -values <0.01 were kept, and we also required that the differences in editing level were higher than 10% between any two samples compared ( Supplementary Table 10 ). We realized that the biological factors causing RNA-editing differences between castes may be complex; hence, we focused on identifying the sites that displayed consistent differences in editing level between two castes across all three different colonies. To identify such consistently differentially edited sites between two castes, we required that these sites satisfied the following two criteria: (i) the caste difference in editing level based on the criteria described in the above paragraph was significant in at least two out of the three colonies, while the third colony showed a difference in the same direction. (ii) The P -values of Fisher’s exact tests using the combined data of the three colonies (that is, pooling the number of reads supporting editing or non-editing across the three colonies) after adjusted by FDR [67] was <0.05. PCR validation of differentially edited sites Three consistently differentially edited sites, targeting CDSs of Aech_08485 (a Zinc finger protein) and the 3′-UTRs of pUf68 and TBPH , were randomly chosen for PCR validation in the nine samples. The nine gDNA and RNA samples for validations were independently collected from the same live lab colonies (Ae322, Ae356 and Ae363) in early 2014 that provided the initial RNA-Seq samples in 2012. Primers are listed in Supplementary Data 6 and validation experiments were performed with the same protocol as described above. Accession codes: DNA resequencing and strand-specific RNA sequencing data of A. echinatior produced in this study as well as the RNA-editing sites identified in the nine A. echinatior samples have been submitted to the NCBI Gene Expression Omnibus (GEO; http://www.ncbi.nlm.nih.gov/geo/ ) under accession number GSE51576 . How to cite this article: Li, Q. et al. Caste-specific RNA editomes in the leaf-cutting ant Acromyrmex echinatior . Nat. Commun. 5:4943 doi: 10.1038/ncomms5943 (2014).